Innate recognition of water bodies in echolocating bats In the course of their lives, most animals must find different specific habitat and microhabitat types for survival and reproduction. Yet, in vertebrates, little is known about the sensory cues that mediate habitat recognition. In free flying bats the echolocation of insect-sized point targets is well understood, whereas how they recognize and classify spatially extended echo targets is currently unknown. In this study, we show how echolocating bats recognize ponds or other water bodies that are crucial for foraging, drinking and orientation. With wild bats of 15 different species (seven genera from three phylogenetically distant, large bat families), we found that bats perceived any extended, echo-acoustically smooth surface to be water, even in the presence of conflicting information from other sensory modalities. In addition, naive juvenile bats that had never before encountered a water body showed spontaneous drinking responses from smooth plates. This provides the first evidence for innate recognition of a habitat cue in a mammal. It is crucial for animals to find their often species-specific, suitable habitat or microhabitat for fitness relevant behaviours, such as mating, breeding, foraging or drinking [1] , [2] . Although both empirical and theoretical work have investigated whether and under which conditions habitat preference is innate or learned [3] , [4] , [5] , [6] , [7] , very little is known about the sensory cues that actually mediate habitat recognition in vertebrates. The only studies known to us show that fish innately find riverine habitats by olfaction [8] and that migrating birds may use song of bird species with similar habitat requirements to find suitable stopover sites [9] . Bats are an especially interesting group in which to study the sensory basis of habitat recognition, because they are highly mobile, can cover 200 km in one night's flight and yet predominantly rely on a short-range sensory system, echolocation [10] . Although it is well understood how bats echolocate insect-sized point targets [10] , [11] , it is unclear how they recognize extended objects such as forest edges or lakes. Ponds, lakes and rivers are important for bats in various ways. They offer an abundance of prey, often soft bodied and easily digestible [12] , and several bat species are specialized to forage in aquatic habitats [13] . Because of acoustic mirror effects, bats can detect insects sitting on the smooth water surface easier [14] , [15] and from further away [16] than on vegetation or when air-borne. With respect to flight costs, bats benefit from the ground effect when flying close to the water surface [17] . Many bat species likely use bodies of water as landmarks for orientation and navigation [18] . Also, most of the about 1,000 extant species of echolocating bats must visit ponds or rivers for drinking ( Fig. 1 ). But how do bats find and recognize the most prominent element of such an aquatic habitat, the water body? Water surfaces are special in that they represent the only extended, acoustically smooth surfaces in the natural environment. We therefore hypothesized that bats would rely on the mirror-like echo reflection properties of smooth water surfaces to detect and recognize bodies of water. When a bat flies over a water surface and the axis of its echolocation beam intersects with the surface at an acute angle, the main energy of the echolocation calls is reflected away from rather than back towards the bat, so it does not receive an echo from ahead ( Fig. 2 ). However, some off-axis energy of the sound beam hits the surface perpendicularly and does generate an echo returning from straight below the bat. On the basis of our above hypothesis, we predicted that bats confronted with any sufficiently large smooth, horizontal surface having these acoustic mirror properties will perceive it to be water. 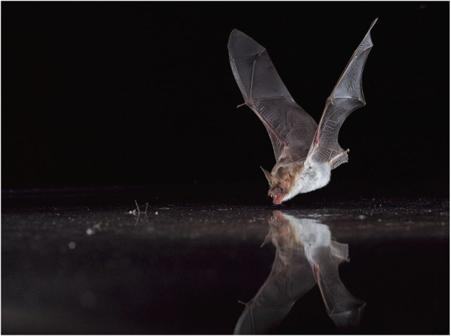Figure 1: Drinking bat. A greater mouse-eared bat,M. myotis, closing in on a water surface, opening its mouth and lowering the head to take a mouthful of water (Photo by Dietmar Nill). Figure 1: Drinking bat. A greater mouse-eared bat, M. myotis , closing in on a water surface, opening its mouth and lowering the head to take a mouthful of water (Photo by Dietmar Nill). 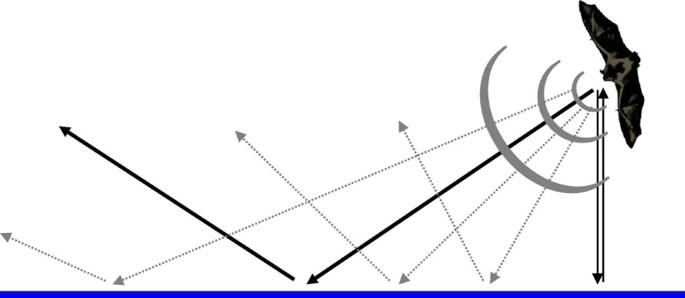Figure 2: Simplified representation of sound propagation and echo generation at a smooth surface. Most of the call energy is reflected away from the bat, with the exception of the small off-axis fraction that hits the surface perpendicularly. Full size image Figure 2: Simplified representation of sound propagation and echo generation at a smooth surface. Most of the call energy is reflected away from the bat, with the exception of the small off-axis fraction that hits the surface perpendicularly. Full size image In this study, we show how free flying bats recognize and classify spatially extended echo targets in an ecologically and evolutionarily relevant context. We took a behavioural approach to find out how bats recognize a key habitat element in their environment: bodies of water. We found that bats take horizontal, acoustical mirrors to be water. This behaviour is extremely stereotypical, phylogenetically widespread among echolocating bats and innate. Echolocation is the key sensory modality triggering water recognition and takes dominance over conflicting information. Echoacoustic water recognition In a large flight room with weak red illumination, we presented experimentally naive, wild-caught bats with two plates (1.2×2 m) positioned on a sandy floor ( Supplementary Fig. S1 ). The two plates presented simultaneously in each trial were always of the same material—either metal, plastic or wood—but one had a smooth and the other a textured surface ( Fig. 3 ). Ensonification and qualitative assessment of the reflected echo scenes showed that the smooth plates were good echoacoustic mimics of a water surface, whereas the echoes of the textured plates resembled those of grained sand ( Fig. 4 ). It is important to note that the smooth experimental plates only mimicked water in the echoacoustic domain, but did not in other modalities, including olfaction, vision, taste and touch. We scored a bat's attempt to drink from an experimental plate as our behavioural measure for the bats' perception of the experimental plate as a water body. To evaluate whether the bats were generally motivated to drink, we presented the bats a real water pool at the end of each experimental session ( Supplementary Fig. S1 ). 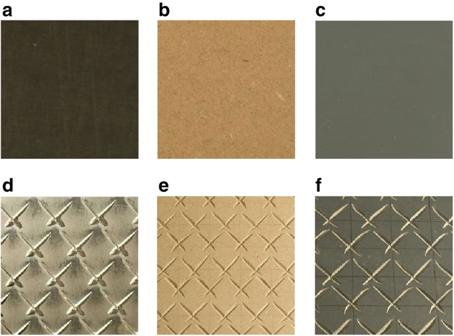Figure 3: Experimental plates. In the first row all smooth surfaces are shown: metal (a), wood (b) and plastic (c); and below the respective textured plates (d–f). Each photo shows a 0.13×0.13 m detail from the 1.2×2 m plates. Figure 3: Experimental plates. In the first row all smooth surfaces are shown: metal ( a ), wood ( b ) and plastic ( c ); and below the respective textured plates ( d – f ). Each photo shows a 0.13×0.13 m detail from the 1.2×2 m plates. 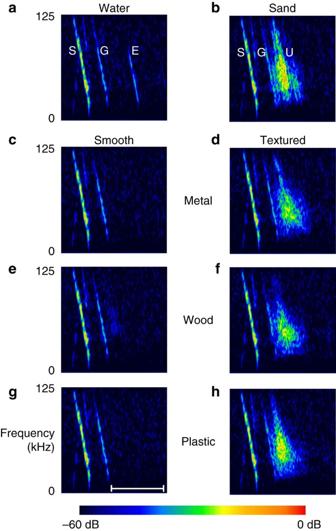Figure 4: Echo signatures of natural and experimental surfaces. In the first row a comparison of a natural smooth (water) (a) and a natural textured surface (sand) (b) is given. Below, the echo signatures of our three experimental materials (metal, wood and plastic) are compared for smooth and textured plates. Smooth plates are depicted on the left (c,e,g) and textured surfaces on the right (d,f,h). The white scale bar ingcorresponds to 10 ms. The colour bar codes for the amplitude of the signal in a relative dB scale.Smooth(left side): After the outgoing signal (S), there is a time delay until the first echo returns; this is the echo front reflected perpendicularly from the ground (G). All other parts of the signal are reflected away and thus do not reach the microphone (seeFig. 2for a schematic representation). In the water sonogram (a), an additional echo from the back edge (E) of the water pool shows up.Textured(right side): After the perpendicular ground echo (G), a series of many overlapping echoes from the uneven surface structures follows (U). Overall, the echo reflections of the smooth experimental plates strongly resemble those of a water surface, whereas the reflections of the textured plates mimic those of uneven ground. Full size image Figure 4: Echo signatures of natural and experimental surfaces. In the first row a comparison of a natural smooth (water) ( a ) and a natural textured surface (sand) ( b ) is given. Below, the echo signatures of our three experimental materials (metal, wood and plastic) are compared for smooth and textured plates. Smooth plates are depicted on the left ( c , e , g ) and textured surfaces on the right ( d , f , h ). The white scale bar in g corresponds to 10 ms. The colour bar codes for the amplitude of the signal in a relative dB scale. Smooth ( left side ): After the outgoing signal (S), there is a time delay until the first echo returns; this is the echo front reflected perpendicularly from the ground (G). All other parts of the signal are reflected away and thus do not reach the microphone (see Fig. 2 for a schematic representation). In the water sonogram ( a ), an additional echo from the back edge (E) of the water pool shows up. Textured ( right side ): After the perpendicular ground echo (G), a series of many overlapping echoes from the uneven surface structures follows (U). Overall, the echo reflections of the smooth experimental plates strongly resemble those of a water surface, whereas the reflections of the textured plates mimic those of uneven ground. Full size image We tested four different species of bat (each n =6 individuals), from distinct ecological [10] and phylogenetic groups [19] with all three plate materials. Schreiber's bat ( Miniopterus schreibersii ) is an example of a species hunting in open space; Daubenton's bat ( Myotis daubentonii ) is specialized at hunting over bodies of water; the greater mouse-eared bat ( Myotis myotis ) forages predominantly for ground-running arthropods; and the greater horseshoe bat ( Rhinolophus ferrumequinum ) uses a distinct and highly specialized echolocation system to detect fluttering insects. All 24 bats of all four species spontaneously tried to drink from the smooth plates of all three materials, but never from the textured plates ( Fig. 5 , Fisher's combined probability test, all P <0.0001). When they were offered a real water pool at the end of each experimental session (control of drinking motivation), they drank 4–19 times in 10 min (species means). To further explore the generality and taxonomic spread of echoacoustic water recognition, we additionally tested one individual from 11 more species with the metal plate setup. Our total data set thus comprises 15 species (7 genera) from 3 large bat families, Vespertilionidae, Miniopteridae and the phylogenetically distant Rhinolophidae [19] . All of the 11 additional species likewise tried to drink from the smooth but never from the textured metal plate ( Table 1 ). 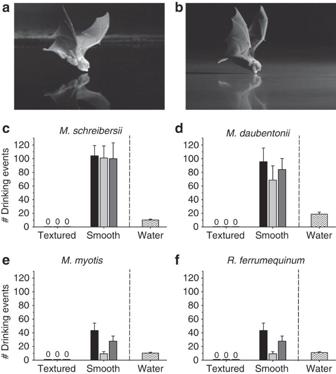Figure 5: Drinking attempts on textured versus smooth surfaces for the four tested bat species. The top panels show aM. schreibersiidrinking from real water (a) and attempting to drink from a metal plate (b). All bats were tested (each speciesn=6) on all three plate materials: metal (black bars), wood (light grey bars) and plastic (dark grey bars). The textured plates are portrayed on the left and marked with a '0', as no drinking attempts occurred. All smooth plates are grouped on the right side. For each species the average drinking events on real water are depicted on the far right. Drinking attempts of (c)M. schreibersii, (d)M. daubentonii, (e)M. myotisand (f)R. ferrumequinum.Error bars show one standard error, for statistics see text. Figure 5: Drinking attempts on textured versus smooth surfaces for the four tested bat species. The top panels show a M. schreibersii drinking from real water ( a ) and attempting to drink from a metal plate ( b ). All bats were tested (each species n =6) on all three plate materials: metal (black bars), wood (light grey bars) and plastic (dark grey bars). The textured plates are portrayed on the left and marked with a '0', as no drinking attempts occurred. All smooth plates are grouped on the right side. For each species the average drinking events on real water are depicted on the far right. Drinking attempts of ( c ) M. schreibersii , ( d ) M. daubentonii , ( e ) M. myotis and ( f ) R. ferrumequinum. Error bars show one standard error, for statistics see text. Full size image Table 1 Drinking attempts of additional bat species. Full size table The bats' behaviour during drinking attempts on the smooth plates and when drinking from the real water was identical (compare Fig. 5a with 5b and Supplementary Movies 1 with 2 ), which shows that the bats indeed tried to drink from the plates. M. schreibersii , the most persistent species, performed an average of 104±15 (mean±s.e.m.) drinking attempts on the smooth metal plate in two 5-min trials ( Fig. 5c ), whereas the other three species reached values of 95±20 ( M. daubentonii ), 47±15 ( M. myotis ) and 43±11 ( R. ferrumequinum ) attempts (analysis of variance, F 1,3 =4.23, P =0.0182). The material of the plates had no effect on the number of drinking attempts in M. schreibersii (repeated measures analysis of variance, F 2,10 =0.01, P =0.9886, Fig. 5c ) and M. daubentonii (F 2,10 =1.06, P =0.3838, Fig. 5d ). By contrast, material type did affect the number of drinking attempts in M. myotis (F 2,10 =4.57, P =0.0389, Fig. 5e ) and R. ferrumequinum (F 2,10 =4.52, P =0.0399, Fig. 5f ). This was driven by a lower response to the wooden plate as compared with metal and plastic. Robustness to conflicting information On rare occasions, bats even resumed their drinking attempts after having accidentally landed on the smooth plate shortly before, whereby they should have perceived that it is not a water body. To further explore the behavioural response of M. schreibersii to an acoustically simulated water surface in a physically unrealistic situation, we placed the metal plate on a table ( Supplementary Fig. S1 ). We were interested to see whether water recognition triggered by the acoustic mirror was imperative enough to override the generated conflict, namely, being able to echolocate underneath a perceived water surface. Some even flew underneath the tabletop. Nevertheless, they repeatedly tried to drink from the metal plate (43±9 attempts in 10 min, n =6 bats), suggesting that water-like echoacoustic cues take dominance over any other conflicting information. In a next step, we evaluated the role of conflicting sensory stimuli with another set of Schreiber's bats. We assume conflicting sensory information in the domains of vision, chemoreception and touch, as a metal plate does not look, smell, taste or feel like real water. We repeated the initially described experiment with two metal plates on the ground, but this time eliminating potentially conflicting visual input by conducting it in complete darkness. Indeed, the number of drinking attempts rose from the previously recorded 104 attempts under red light conditions to 166 in darkness ( t -test, t 10 =2.48, P =0.0325), whereas the number of drinking events with real water did not differ between the two illumination treatments ( t 10 =1.25, P =0.2408) ( Fig. 6a ). 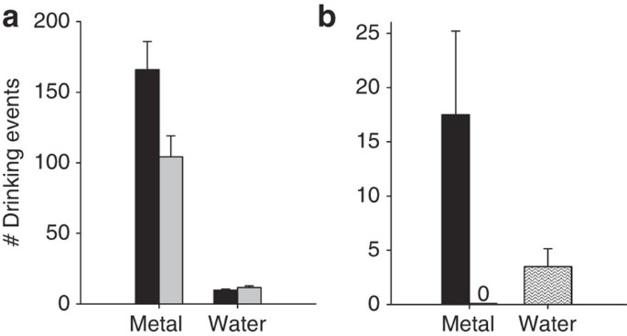Figure 6: Sensory conflict and innate water recognition. In further experiments we examined the role of conflicting information and an innate basis of water recognition. Error bars show one standard error, for statistics see text. (a) Drinking attempts of Schreiber's bat,M. schreibersii(n=6) on a smooth metal plate in different light conditions. No attempts occurred on the simultaneously present textured plate (data not shown). The bats tried to drink significantly more often in complete darkness (black bars) compared with the dim light condition (light grey bars). The drinking numbers on real water did not differ between the two treatments. (b) Drinking attempts of naive, juvenile Geoffroy's bats,M. emarginatus(n=6), from metal plates (black bars). Not a single attempt occurred on the textured plate, thus marked with a '0'. On the right the number of drinking events on real water is shown. Figure 6: Sensory conflict and innate water recognition. In further experiments we examined the role of conflicting information and an innate basis of water recognition. Error bars show one standard error, for statistics see text. ( a ) Drinking attempts of Schreiber's bat, M. schreibersii ( n =6) on a smooth metal plate in different light conditions. No attempts occurred on the simultaneously present textured plate (data not shown). The bats tried to drink significantly more often in complete darkness (black bars) compared with the dim light condition (light grey bars). The drinking numbers on real water did not differ between the two treatments. ( b ) Drinking attempts of naive, juvenile Geoffroy's bats, M. emarginatus ( n =6), from metal plates (black bars). Not a single attempt occurred on the textured plate, thus marked with a '0'. On the right the number of drinking events on real water is shown. Full size image Innate response of juvenile bats Bats are able to efficiently learn from conspecifics [20] , but they typically roam and forage alone [21] , [22] . We thus hypothesized that echoacoustic recognition of water surfaces would most likely be innate. To test this hypothesis, we raised six juvenile Geoffroy's bats ( M. emarginatus ) at our field station together with their mothers. They were captured in a cave before they became volant and hence had never encountered a pond or river in their life. As soon as they flew well, these naive bats were tested with the metal plate setup. Five of the six juveniles, on this first contact in their life with an extended, horizontal smooth surface, spontaneously tried to drink from the smooth metal plate (18±8 times; Fig. 6b ), but never from the textured plate (Fisher's combined probability test, P <0.0001, n =6 bats). The juvenile drinking attempts very much resembled those observed in the adults. The one juvenile bat that did not attempt to drink from the metal plate also did not drink from the subsequently presented real water and thus probably lacked sufficient motivation. The behavioural data corroborate our hypothesis that bats rely on the mirror-like echo reflection properties of smooth water surfaces to detect and recognize water bodies. It is astonishing that all individuals attempted to drink repeatedly, some even 100 times and more, from the plates with the water-like echo signature, despite conflicting information from other sensory modalities, such as touch, taste, olfaction and vision. This suggests that bats rely heavily on echolocation for assessment of their environment at close range and for the recognition of habitat elements. The observation that all 15 species, representative for three large and phylogenetically distant bat families, very reproducibly showed drinking attempts on large smooth plates furthermore suggests that echoacoustic water recognition is taxonomically wide spread, if not universal, among echolocating bats. The high number of consecutive drinking attempts that the bats showed within a short time, despite being unsuccessful, indicates a hardwired neural processing of echoacoustic water recognition. However, the fact that two species showed fewer attempts on the wooden than on the metal and plastic plates indicates that other modalities also had some inferior role. Possibly, the light wooden plates were visually most dissimilar from water or had the most distinct non-water smell, and the conflicting information of these modalities lowered the bats' behavioural response. By conducting the experiment with M. schreibersii again in complete darkness, we removed the conflicting visual information and thereby altered the sensory scenery. We observed an increase of drinking attempts by almost 60% in complete darkness. As the drinking events on real water after the experiment stayed on the same level as before, this is not the result of a potential side effect due to increased drinking motivation. Our experiments suggest that the bats integrate information from several modalities to form a percept of their environment [23] and to inform their behavioural decisions. However, cue importance in this weighted sensory integration process seems to be heavily biased towards echoacoustic information, given that the echoacoustic illusion was sufficient to make bats perceive a water surface. Merely the robustness of this percept could be slightly modulated by other sensory modalities. With respect to small-scale navigation [10] and habitat recognition, bats thus appear to be an extreme example of predominant reliance on one main sensory modality. For large-scale navigation—where echolocation has a much smaller role [10] —bats use and integrate information across modalities, such as visual and magnetoreceptive information [24] . The present extreme case of one sensory input's prevalence might be an interesting model to further increase the current understanding of multisensory integration in the vertebrate brain [25] , [26] . To date, many other multimodal studies—often focused on communication—found a more balanced integration of multisensory stimuli. Communicating dart-poison frogs, for example, require concurrent visual and auditory cues for cross-modal integration to elicit a behavioural response [27] . With the bats' response being so extremely stereotypical and repetitive, questions about learning arise. Do bats have to learn water recognition by following conspecifics, for example, their mother? The answer is no. By contrast, the spontaneous and repeated drinking attempts of the juvenile, naive bats strongly argue for an innate basis of the echoacoustic recognition of water bodies. Given that bats mistake large horizontal mirrors innately and persistently for water, one might hypothesize that they occasionally try to drink from man-made smooth surfaces, such as car roofs, winter gardens and the like. Future studies will be necessary to assess the occurrence, extent and potential conservation relevance of such a scenario. Certainly, bats also need to recognize other specific foraging habitats to which the respective species are adapted in, for example, wing morphology, echolocation system and food requirements [10] , [28] , [29] , [30] . Computers can classify tree species on the basis of echo statistics [31] —so bats may as well. Bats can distinguish the roughness of computer-generated echoes [32] ; an ability that might help them classifying complex vegetation echoes. From a technical perspective, a detailed understanding of how bats echolocate and recognize spatially extended objects and habitat types will further the development of sonar-based autonomous robots. In summary, our experiments revealed that the recognition of water bodies in bats is mediated by echoacoustic cues (mirror-like reflection). This recognition mechanism is taxonomically wide spread among bats, and our experiments strongly suggest it is innate. To our knowledge, this is the first example of innate recognition of a habitat cue in mammals. The innateness and the physically well-defined cues make water recognition in bats an ideal model to study the neural basis and potentially even the genetic correlates of habitat recognition. Bats This study was conducted at the Tabachka Bat Research Station of the Sensory Ecology Group (Max Planck Institute for Ornithology, Seewiesen), which is run in cooperation with the Directorate of the Rusenski Lom Nature Park in the district of Ruse, northern Bulgaria. Capture, husbandry and behavioural studies were carried out under license of the responsible Bulgarian authorities (Bulgarian Ministry of Environment and Water and Regional Inspectorate (RIOSV) Ruse, permits # 57/18.04.2006 and 100/04.07.2007). Bats were captured in the area of the Rusenski Lom Nature Park at or close to their roost caves by a handnet, mistnets or harp trap. For the duration of the experiment, bats were kept in a separate keeping room (temperature 18–24 °C, humidity around 75%; close to natural conditions in the caves, own data). Depending on the species, they were accommodated in either a 2.2×0.9×1.1 m mesh tent or 50×35×35 cm cages. On the capture night, bats were handfed with mealworms and watered until satiated. The experiment was usually started on the following night. All bats were released again at their respective capture site after completion of the experiment. Four species of bat were used for the full set of the experiments with all three plate materials (metal, plastic and wood): M. schreibersii , M. daubentonii , M. myotis and R. ferrumequinum . Six adult individuals per species were tested in a balanced sex ratio. To test for the generality and the extent of the taxonomic spread of our findings, 1 individual each from 11 additional bat species was tested with the metal plate setting (see below). This group consisted of Myotis emarginatus , M. nattereri , M. capaccinii , M. blythii oxygnathus , M. bechsteinii , M. aurascens , Hypsugo savii , Plecotus austriacus , Nyctalus noctula , Pipistrellus pipistrellus and Rhinolophus mehelyi . Six females of the Geoffroy's bat ( M. emarginatus ) were captured inside a cave with their young shortly before those became volant. Mothers were kept with the juveniles and nursed them until natural weaning. When released together into their home cave after completion of experiments, the juveniles were able to fly and forage independently. Six additional adult M. schreibersii were used to test their drinking response in complete darkness (dark condition). Flight room and experimental setup All experiments were conducted in a large flight room (4×8×2.4 m). The floor was covered with sand, and the walls and ceiling with a felt-like, sound-dampening material ('Velter', thickness 5 mm, Arbanasy EOOD). The room was lit with two red bulbs (25 W, Osram), except for the dark condition (see below), where custom-made infrared strobe lights (Animal Physiology Department, University of Tübingen, Germany; 875 nm wavelength) were used. In the centre of the room, a water pool was inserted into the sandy floor (1.8×1 m, 4 cm water depths) ( Supplementary Fig. S1 ). The pool could be covered by a plate and sand, or uncovered to give the bats access to real water. To test our hypothesis that the bats would take any extended, acoustically smooth horizontal surface for water, we presented experimental plates (1.2×2 m) on the flight room floor. Always two plates of the same material but with different surface structure (one smooth, one textured) were presented side by side in the centre of the flight room (25 cm distance between plates; pool covered) ( Supplementary Fig. S1 ). We used three different materials for the experimental plates: metal (aluminium), plastic (polyvinyl chloride) and wood (medium-density fibreboard). For the textured surfaces, we chose a metal diamond plate with 35×5 mm ( ∼ 2 mm height) bumps at 4 cm spacing, while we carved depressions of the same size and spacing into the plastic and wooden plates (see Fig. 3 ). The bats' behaviour was filmed with four synchronized video cameras (Watec, WAT-902H2 Ultimate; two for overview, two for close-up at the two experimental plates on the ground) for online observation from an adjacent room and for later off-line analysis (ABUS Security Center; Digi-Protect Video Surveillance PCI Card, 4 channel/100 fps). In addition, a high-speed camera (Mikrotron MotionBLITZ EoSens mini) was used for detailed comparison of drinking behaviour from real water with attempts to drink from the smooth experimental plates. Experimental procedure Experiments were conducted at night during the natural activity phase of the bats. The night before the experiment, bats were fed and watered until satisfied. They had access to food and water ad libitum for the rest of the pre-experimental night. Water was taken away in the morning to prevent drinking during the day and early evening. We thereby mimicked natural conditions and thirst levels of bats emerging from their day roosts at dusk. Before each experiment, the bat was fed three to five mealworms. It was then released into the flight room where a smooth and a textured experimental plate were presented. If a bat did not fly and explore the flight room within 1 h, it was excluded from the experiment (total of 19 bats). All other bats attempted to drink from the plates within 1 h. With the first attempt a 5-min time window (time in flight) opened, during which the drinking attempts were counted in later off-line video analysis. We defined a drinking attempt as the bat touching the plate in a head-down position, which corresponds to drinking behaviour from a real water surface (compare Supplementary Movies 1 and 2 ). After these 5 min, the plate positions were exchanged. Again, the bat was given 1 h, and when it resumed drinking attempts, a second 5-min time window began, during which attempts were counted. With completion of this time slot, the plates were removed from the room and the water pool was uncovered. This was performed to assess whether the bat was indeed motivated to drink. It was given one final hour, with a 10-min time window starting as soon as the bat began to drink. All drinking events were counted. During all these trials the bat was free to fly around and explore the room. However, when a bat hung without moving longer than about 3 min, the experimenter went inside to gently stimulate flight by, for example, tapping on the wall. This was performed to prevent the bat from falling asleep. After the experiment, the bat was fed and watered until satisfied, and then returned to its keeping cage. In the two consecutive nights, the experiment was repeated with the remaining two substrate types. To factor out effects of presentation sequence, the three plate materials (metal, plastic and wood) were assigned to nights and bats following a Latin square design. To test for the persistence of the bats' drinking response in a physically unrealistic situation for a pond or river, the metal plate was placed on a standard plastic garden table (1.5×1 m, 1 m height) in a way that the bats could assess the open airspace below the tabletop by echolocation and fly underneath ( Supplementary Fig. S1 ). The M. emarginatus juveniles received regular flight training in the empty flight room to ensure natural development of flight abilities. Once fully volant, they were tested individually in the metal plate setup as described above for the adult bats. Also the test of the six additional adult M. schreibersii in the dark condition (metal plates only) followed all experimental details as previously described, with the exception that infrared light was used instead of dim red light (see above). Data analysis Statistical analyses were run in SPSS 15.0 and Excel 2003. Because all tested bats showed zero drinking attempts for all of the textured plates, we refrained from using parametric tests for an assessment of surface structure on the bats' behaviour. Instead, we computed separate χ 2 -tests to compare the number of drinking attempts for the smooth versus the textured plates for each bat and plate material. From these, we calculated combined P -values using Fisher's combined probability test. Ensonification For qualitative evaluation of the echo scenes reflected back by the experimental plates, by real water and a sand surface, we ensonified these surfaces with an artificial echolocation call created in Adobe Audition, sweeping from 120 down to 20 kHz with 3 ms duration (results given in Fig. 4 ). This artificial call encompasses the main frequency range used by all tested bat species. The call was played by a Polaroid loudspeaker and amplifier (custom-made, University of Tübingen, Germany), which was connected through a PCMCIA card (DAQ Card 6062E, National Instruments) with a computer running Avisoft (Avisoft Bioacoustics) software. Returning echoes were recorded by an Avisoft microphone (Type CM16/CMPA, Avisoft Bioacoustics) by an ultrasound recording interface (UltraSoundGate 416H, Avisoft Bioacoustics) and using Avisoft recording software (Avisoft Recorder USGH) with 500 kHz sampling rate. Speaker and microphone on top were mounted in parallel 62 cm above the ensonified surface and tilted downwards in a way that the speaker's acoustic axis intersected with the surface at an angle of 50°. How to cite this article: Greif, S. & Siemers B. M. Innate recognition of water bodies in echolocating bats. Nat. Commun. 1:107 doi: 10.1038/ncomms1110 (2010).